Light-inducible receptor tyrosine kinases that regulate neurotrophin signalling Receptor tyrosine kinases (RTKs) are a family of cell-surface receptors that have a key role in regulating critical cellular processes. Here, to understand and precisely control RTK signalling, we report the development of a genetically encoded, photoactivatable Trk (tropomyosin-related kinase) family of RTKs using a light-responsive module based on Arabidopsis thaliana cryptochrome 2. Blue-light stimulation (488 nm) of mammalian cells harbouring these receptors robustly upregulates canonical Trk signalling. A single light stimulus triggers transient signalling activation, which is reversibly tuned by repetitive delivery of blue-light pulses. In addition, the light-provoked process is induced in a spatially restricted and cell-specific manner. A prolonged patterned illumination causes sustained activation of extracellular signal-regulated kinase and promotes neurite outgrowth in a neuronal cell line, and induces filopodia formation in rat hippocampal neurons. These light-controllable receptors are expected to create experimental opportunities to spatiotemporally manipulate many biological processes both in vitro and in vivo . Cells respond to their environment by transducing external stimuli, for example growth factors and hormones, into relevant internal signals via cell-surface receptors, such as G-protein-coupled receptors [1] and receptor tyrosine kinases (RTKs) [2] . By binding to their ligands, receptors mediate the activation of diverse intracellular signalling pathways and regulate numerous cellular processes. Accordingly, natural ligands or synthetic agonists have been broadly used as indispensable tools to specifically control receptor activity and probe the mechanisms underlying cellular behaviours. However, they do not allow spatial control and have temporal resolution that is limited by time required for diffusion, making it difficult or impossible to dissect and analyse the dynamic nature of cellular signalling networks in a spatiotemporally precise manner. One promising approach to circumvent these limitations is coupling light signals to receptor activity. Because the activating stimulus (light) can be delivered with high spatiotemporal specificity, and even simply switched on and off, experimental opportunities are created that would not be possible with classical ligand-based and pharmacological methods. To date, efforts to control cell signalling through optical modulation of receptor activity have mainly used vertebrate rhodopsin, as exemplified by engineered chimeric receptors that combine rhodopsin with G-protein-coupled receptors [3] , [4] . Recently developed light-responsive interacting modules [5] , [6] , [7] may represent a new strategy for light activation of receptors. The members of a module pair, which are based on plant photoreceptors derived from Arabidopsis thaliana , are genetically encoded and allow control of protein–protein interactions in mammalian cells in a light-dependent fashion, thereby suitable for application to receptor systems that are activated by an interaction between receptor monomers, such as RTKs. Normally, RTK activation is induced by ligand-mediated receptor dimerization ( Fig. 1a ), which in turn leads to autophosphorylation of tyrosine kinase domains and recruitment of downstream signalling molecules [2] . However, this interaction, and thus receptor activation, can be induced artificially using chemical inducers of dimerization (CIDs) [8] . In this application, tyrosine kinase domains are fused to the binding domain(s) recognized by CIDs, allowing RTKs to be pharmacologically crosslinked and activated, independently of their endogenous counterpart and ligand, in the presence of CIDs such as rapamycin or AP20187 (refs 9 , 10 , 11 ). Accordingly, we reasoned that the light-mediated interactions could functionally substitute for the CID approach and allow RTKs to be dimerized and activated in response to light. 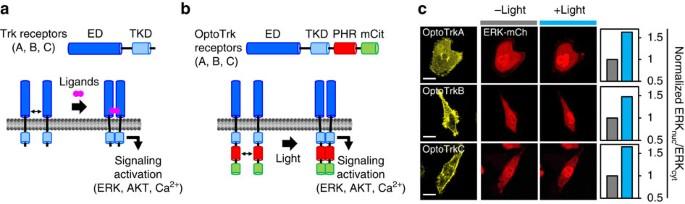Figure 1: Design and functional expression of photoactivatable Trk receptors. Schematic illustration of the molecular architecture and activation process of (a) Trk and (b) optoTrk receptors. Sites of induced monomer interaction are denoted by left right arrows. ED, extracellular domain; TKD, tyrosine kinase domain; and mCit, mCitrine. (c) Fluorescence images of optoTrk receptors and ERK-mCherry co-expressed in HeLa cells. ERK-mCherry (ERK-mCh) was imaged before and 5 min after a single-light stimulation (488 nm, three 0.5-s pulses, 6.5 μW). Graphs on the right show the normalized ratio of nucleus and cytosol ERK-mCh fluorescence (ERKnuc/ERKcyt) before (grey bar) and after (blue bar) blue-light exposure. Scale bars, 20 μm. Figure 1: Design and functional expression of photoactivatable Trk receptors. Schematic illustration of the molecular architecture and activation process of ( a ) Trk and ( b ) optoTrk receptors. Sites of induced monomer interaction are denoted by left right arrows. ED, extracellular domain; TKD, tyrosine kinase domain; and mCit, mCitrine. ( c ) Fluorescence images of optoTrk receptors and ERK-mCherry co-expressed in HeLa cells. ERK-mCherry (ERK-mCh) was imaged before and 5 min after a single-light stimulation (488 nm, three 0.5-s pulses, 6.5 μW). Graphs on the right show the normalized ratio of nucleus and cytosol ERK-mCh fluorescence (ERK nuc /ERK cyt ) before (grey bar) and after (blue bar) blue-light exposure. Scale bars, 20 μm. Full size image In this study, our goal was to develop photoactivatable RTKs. The tropomyosin-related kinase (Trk) family was chosen as a candidate light-induced RTK. Following binding to neurotrophins, the three members of this family, Trk A, B and C, mediate activation of intracellular signalling pathways, including mitogen-activated protein kinase kinase (MEK)/extracellular signal-regulated kinase (ERK), phosphatidylinositol 3-kinase (PI3K)/Akt and phospholipase Cγ1 (PLCγ1)/Ca 2+ pathways, and thereby contribute to neuronal survival, neurite outgrowth and synaptic plasticity [12] . As a light-inducible dimerization system, we initially introduced the photolyase homology region (PHR) of cryptochrome 2, a blue-light photoreceptor, and its optically driven interaction partner CIBN, an N-terminal domain of CIB1, because the PHR-CIBN pair achieves fast and precise control of protein–protein interactions upon blue-light exposure with no requirements for exogenous cofactors [7] . However, we unexpectedly found that PHR can be harnessed as a homo-interaction domain to activate the linked Trk receptors in response to light ( Fig. 1 and Supplementary Fig. 1 ). Exploiting this serendipitous outcome, we were able to achieve optically activatable Trk signalling using a single light-responsive module ( Fig. 1b ). Here we show that light stimulation can activate canonical Trk signalling pathways through photoactivatable Trk receptors, designated optoTrks. Using one of the receptors, optoTrkB, we representatively show that TrkB signalling is rapidly and transiently controlled by a single photostimulation in a reversible, spatial and cell-specific manner. In addition, a prolonged patterned stimulation (illumination) of a neuronal cell line harbouring optoTrkB sustains ERK activity and induces neuronal differentiation. Finally, we further demonstrate the utility of optoTrk receptors by showing that blue-light exposure can trigger PI3K signalling activation and regulate neurite outgrowth, as well as filopodia formation in rat hippocampal neurons. Design of optoTrk receptors As schematically illustrated in Supplementary Fig. 1a , we originally designed two different chimeric receptors containing full-length Trk, one consisting of Trk linked to PHR and the monomeric yellow fluorescent protein mCitrine (Trk-PHR-mCit), and the other consisting of Trk linked to CIBN and the monomeric cyan fluorescent protein mCerulean (Trk-CIBN-mCer). To test the PHR-CIBN interaction-mediated activation of Trk signalling in mammalian cells, we first constructed PHR- and CIBN-fused TrkB receptors and expressed them together or individually in PC12 or HeLa cells, both of which do not express endogenous TrkB receptors [13] , [14] . Illumination of cotransfected PC12 cells using a blue LED array (470 nm, 5.5 μW) caused an increase in endogenous phospho-ERK level ( Supplementary Fig. 1b ), suggesting a light-induced activation of ERK signalling. Unexpectedly, we found that TrkB-PHR-mCit alone was able to activate ERK in response to light stimulation, whereas TrkB-CIBN-mCer was not ( Supplementary Fig. 1b ). To further verify this phenomenon, we imaged intracellular Ca 2+ level ([Ca 2+ ] i ). Exposure of HeLa cells harbouring both of the two chimeric receptors to blue-light stimulation (488 nm, three 0.5 s pulses, 6.5 μW) evoked a Ca 2+ transient, as demonstrated by an increase in the fluorescence intensity of cotransfected, intensiometric Ca 2+ indicator (R-GECO1) [15] shown in Supplementary Fig. 1c . Again, TrkB-PHR-mCit alone was sufficient to drive changes in [Ca 2+ ] i in response to blue-light pulses, whereas TrkB-CIBN-mCit, mCitrine-tagged TrkB (TrkB-mCit), or mCitrine-tagged PHR (PHR-mCit) did not elevate [Ca 2+ ] i after light stimulation ( Supplementary Fig. 1c ). Moreover, we did not observe light-triggered Ca 2+ signal when TrkB receptor linked to a light-insensitive PHR mutant (PHR D387A ) [16] (TrkB-PHR D387A -mCit) was expressed ( Supplementary Fig. 1c ). Collectively, these results suggested that the PHR domain alone is able to confer a light-inducible interaction capacity on the linked TrkB receptor, thereby allowing it to mediate ERK and Ca 2+ signalling in response to light. Thus, using a single light-dependent homo-interaction domain, we were able to construct a photoactivatable TrkB receptor, designated optoTrkB ( Fig. 1b ). Extending this concept to other members of the Trk family, we also constructed photoactivatable TrkA and TrkC receptors, optoTrkA and C ( Fig. 1b ). Light-induced upregulation of canonical Trk signalling To validate functional expression of optoTrks, we used biosensors of intracellular ERK, AKT and Ca 2+ signalling activity to assay light-induced activation of canonical Trk signalling cascades in individual HeLa cells by live-cell imaging. Blue-light illumination of cells transfected with each optoTrk receptor clearly caused nuclear translocation of monomeric (m)Cherry-tagged ERK (ERK-mCh), indicating ERK pathway activation [17] ( Fig. 1c ). In addition, light stimulation promoted plasma membrane localization of the pleckstrin homology domain of mCherry-tagged AKT1 (mCh-PH AKT1 ) ( Supplementary Fig. 2a ), indicating PI3K/Akt signalling activation [18] , and resulted in an increase in R-GECO1 signal, demonstrating [Ca 2+ ] i elevation ( Supplementary Fig. 2b ). Taken together, these results indicate that optoTrk receptors can induce upregulation of ERK, AKT and Ca 2+ signalling pathways upon blue-light exposure. Among the modified receptors, we used optoTrkB for all follow-up studies. Differential regulation of TrkB signalling by BDNF and light TrkB signalling is activated by binding of TrkB receptor to its cognate ligand brain-derived neurotrophic factor (BDNF) [19] , and the BDNF-binding sites within optoTrkB remain intact. Thus, to characterize the light-triggered activation of TrkB signalling cascades in more detail, we co-expressed optoTrkB with ERK-, PI3K- and Ca 2+ -biosensors, and monitored and analysed their responses to BDNF or blue-light stimulation in a time-dependent manner. At first, both stimuli caused an increase of ERK-mCh in the cell nucleus ( Fig. 2a ) and an accumulation of mCh-PH AKT1 at the plasma membrane ( Fig. 2b ). Kinetic measurements of ERK-mCh and mCh-PH AKT1 translocation, however, revealed a common, stimulus-dependent difference: BDNF (50 ng ml −1 ) induced relatively slow, sustained signalling activation in optoTrkB-expressing cells during the examined periods ( Fig. 2a–c ), whereas blue light triggered rapid, transient responses ( Fig. 2a–c ). For example, the normalized nucleus/cytosol ratio of ERK-mCh was gradually increased and maintained at the elevated level, at least until 20 min, in the presence of BDNF, but it was rapidly increased and declined to the baseline after a single light stimulation ( Fig. 2c ). Changes in ERK phosphorylation states, revealed by an immunoblot analysis, after applying the two stimuli were also consistent with this observation ( Supplementary Fig. 3 ). 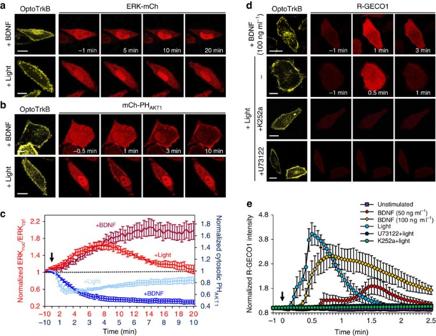Figure 2: BDNF and light stimulation differentially affected on TrkB signalling kinetics. Time-lapse images showing (a) nuclear translocation of ERK-mCh and (b) plasma membrane recruitment of mCh-PHAKT1in response to stimulation of optoTrkB-cotransfected HeLa cells with BDNF (50 ng ml−1) or blue light (three 0.5-s pulses, 6.5 μW). OptoTrkB expression is shown on the left. Scale bars, 20 μm. (c) Translocation kinetics of ERK-mCh and mCh-PHAKT1after stimulation (arrow) of optoTrkB-cotransfected HeLa cells with BDNF or blue light. The graph shows quantified translocation by calculating the ratio of nuclear to cytosolic ERK-mCh (ERKnuc/ERKcyt) and changes in cytosolic mCh-PHAKT1, each normalized to baseline (at −1 min; dotted lines). Coloured numbers on each axis of the graph display different timescales and fold-change scales between ERK-mCh (red) and mCh-PHAKT1(blue) translocation. Error bars, ±s.e.m. (n>8). (d) Time course of changes in R-GECO1 fluorescence in HeLa cells expressing the indicated constructs before and after exposure to BDNF (100 ng ml−1) or light. Cells were photostimulated with or without a 30-min pre-incubation with 100 nM K252a or 2.5 μM U73122. Scale bars, 20 μm. (e) Ca2+signalling kinetics in HeLa transfected and stimulated as ind. Intracellular Ca2+levels were quantified as changes in R-GECO1 fluorescence intensity divided by baseline fluorescence (at −1 min). Error bars, ±s.e.m. (n>8). Figure 2: BDNF and light stimulation differentially affected on TrkB signalling kinetics. Time-lapse images showing ( a ) nuclear translocation of ERK-mCh and ( b ) plasma membrane recruitment of mCh-PH AKT1 in response to stimulation of optoTrkB-cotransfected HeLa cells with BDNF (50 ng ml −1 ) or blue light (three 0.5-s pulses, 6.5 μW). OptoTrkB expression is shown on the left. Scale bars, 20 μm. ( c ) Translocation kinetics of ERK-mCh and mCh-PH AKT1 after stimulation (arrow) of optoTrkB-cotransfected HeLa cells with BDNF or blue light. The graph shows quantified translocation by calculating the ratio of nuclear to cytosolic ERK-mCh (ERK nuc /ERK cyt ) and changes in cytosolic mCh-PH AKT1 , each normalized to baseline (at −1 min; dotted lines). Coloured numbers on each axis of the graph display different timescales and fold-change scales between ERK-mCh (red) and mCh-PH AKT1 (blue) translocation. Error bars, ±s.e.m. ( n >8). ( d ) Time course of changes in R-GECO1 fluorescence in HeLa cells expressing the indicated constructs before and after exposure to BDNF (100 ng ml −1 ) or light. Cells were photostimulated with or without a 30-min pre-incubation with 100 nM K252a or 2.5 μM U73122. Scale bars, 20 μm. ( e ) Ca 2+ signalling kinetics in HeLa transfected and stimulated as in d . Intracellular Ca 2+ levels were quantified as changes in R-GECO1 fluorescence intensity divided by baseline fluorescence (at −1 min). Error bars, ±s.e.m. ( n >8). Full size image Ca 2+ signalling kinetics showed a similar difference between the two stimuli. [Ca 2+ ] i elevation by BDNF (100 ng ml −1 ) was induced slowly and sustained above the basal level for >2 min, whereas light-provoked Ca 2+ transients was rapidly developed and disappeared within 90 s ( Fig. 2d,e ). The slow kinetics of TrkB signalling induced by activation with BDNF was attributable, in part, to the time required for BDNF diffusion and the concentration used. For example, doubling the amount of BDNF from 50 to 100 ng ml −1 shortened the time to the onset of a Ca 2+ surge (defined as a 50% increase in [Ca 2+ ] i above baseline) from 67.9±7.6 to as little as 27±3.3 s (mean±s.e.m. ; Fig. 2e ). Light stimulation caused a much faster Ca 2+ surge (within 17.6±3.1 s (mean±s.e.m. ); Fig. 2e ), demonstrating the much greater temporal resolution of optically activated TrkB signalling. In contrast to responses to BDNF, which were somewhat sustained, responses to light stimulation of optoTrkB were short-lived and rapidly recovered to baseline. This was true for ERK and AKT activity ( Fig. 2a–c ), as well as changes in [Ca 2+ ] i ( Fig. 2d,e ). In addition, when we compared the optoTrkB performance by light with wild-type TrkB receptor activity by BDNF, similar differences in signalling activation kinetics were observed ( Supplementary Fig. 4a–d ). Taken together, these observations suggest that optoTrkB enables transient activation of the canonical TrkB signalling by a single photostimulation. Signalling specificity of optoTrkB We investigated the signalling specificity of optoTrkB. Light-induced ERK activation was totally eliminated by PD0325901, a MEK inhibitor ( Supplementary Fig. 5a ). In addition, LY294002, a PI3K inhibitor, and U73122, a PLC inhibitor, completely blocked light-mediated translocation of mCherry-PH AKT1 to the plasma membrane ( Supplementary Fig. 5b ) and light-triggered [Ca 2+ ] i elevation ( Fig. 2d,e ), respectively. Notably, those light-driven responses were abolished by K252a, a selective inhibitor of Trk tyrosine kinase activity ( Supplementary Fig. 5 and Fig. 2d,e ). These results indicate that the stimulatory effect of blue light on cells expressing optoTrkB is mediated through specific signalling cascades emanating from TrkB activation. Versatile control of TrkB signalling using optoTrkB We postulated that it would be feasible to achieve versatile control of light-gated TrkB signalling by manipulating illumination methods. To explore this, we took advantage of the fast response and recovery time (<90 s from activation to recovery; Fig. 2e ) and simple readout of Ca 2+ imaging. Exposure of HeLa cells cotransfected with optoTrkB and R-GECO1 to initial three 0.5-s blue-light pulses induced a rapid increase and subsequent decline in R-GECO1 fluorescence. After a 10-min interstimulus interval (ISI), a second photostimulation caused a change in intensity similar to that of the first stimulation ( Fig. 3a,b and Supplementary Movie 1 ), demonstrating that this process can be controlled in a reversible manner. We further investigated the reversibility efficacy (defined as the ratio of the second peak amplitude to the first peak amplitude) of light-switched activation of TrkB-PLCγ1-Ca 2+ signalling by varying ISIs. At ISIs of or longer than 5 min (5 and 10 min), a second Ca 2+ transient was evoked with little or no loss of efficacy, whereas at ISIs shorter than 5 min (4 and 3 min), a second stimulus elicited a reduced response in a stepwise fashion ( Fig. 3c and Supplementary Fig. 6 ). And, delivery of two light stimuli spaced 2 min apart did not induce a second Ca 2+ signal ( Fig. 3c and Supplementary Fig. 6 ), overall suggesting a linear relationship between ISI and reversibility efficacy. Based on these results, we could repeatedly generate robust [Ca 2+ ] i elevations (at least five times) in a single cell with a train of blue-light pulses at a constant ISI (10 min) ( Fig. 3d ). 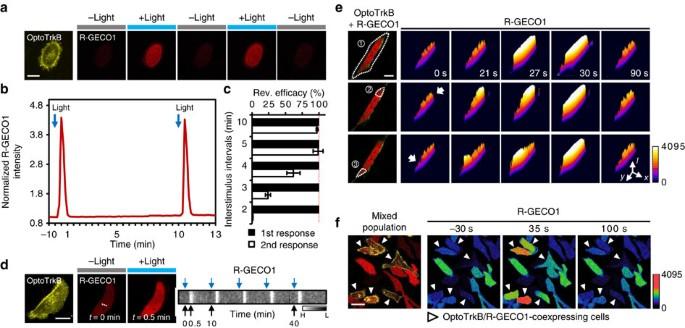Figure 3: Versatile modulation of TrkB signalling using light. (a) Fluorescence images of HeLa cells expressing the indicated constructs before and after delivery of three 0.5-s pulses of blue light (6.5 μW) twice with a 10-min interstimulus interval (ISI). Scale bar, 20 μm. (b) A normalized trajectory of changes in R-GECO1 fluorescence for the cell shown ina. Arrows indicate stimulation. (c) Relationship between reversibility (rev.) efficacy and ISI. Rev. efficacy was determined as the ratio of the normalized second peak R-GECO1 fluorescence (white bars) to the normalized first peak (black bars), expressed as a percentage, in each cotransfected HeLa cells stimulated twice with blue-light pulses with varying ISIs. Error bars, ±s.e.m. (n>7). (d) (Left) Fluorescence images of a HeLa cell expressing the indicated constructs before and 0.5 min after blue-light exposure. Scale bar, 20 μm. (Right) Kymograph drawn along the white dashed line within the cell shown on the left. The cell was illuminated five times (blue arrows above the kymograph) every 10 min. (e) (Left) A HeLa cell co-expressing optoTrkB and R-GECO1 was exposed to whole-cell () or local ( and ) light stimulation. The stimulated areas are outlined with white dashed lines. (Right) Time-lapse, pseudocolored surface intensity plots. Local stimulation is marked with arrows. Axis labelled ‘I’ represents intensity. Scale bar, 20 μm. (f) Selective induction of Ca2+transients. HeLa cells transfected with R-GECO1 or cotransfected with optoTrkB and R-GECO1 (arrowheads) were co-cultured (mixed population) and simultaneously exposed to blue-light pulses. Time courses of R-GECO1 responses are represented by ratio images. Scale bar, 50 μm. Figure 3: Versatile modulation of TrkB signalling using light. ( a ) Fluorescence images of HeLa cells expressing the indicated constructs before and after delivery of three 0.5-s pulses of blue light (6.5 μW) twice with a 10-min interstimulus interval (ISI). Scale bar, 20 μm. ( b ) A normalized trajectory of changes in R-GECO1 fluorescence for the cell shown in a . Arrows indicate stimulation. ( c ) Relationship between reversibility (rev.) efficacy and ISI. Rev. efficacy was determined as the ratio of the normalized second peak R-GECO1 fluorescence (white bars) to the normalized first peak (black bars), expressed as a percentage, in each cotransfected HeLa cells stimulated twice with blue-light pulses with varying ISIs. Error bars, ±s.e.m. ( n >7). ( d ) (Left) Fluorescence images of a HeLa cell expressing the indicated constructs before and 0.5 min after blue-light exposure. Scale bar, 20 μm. (Right) Kymograph drawn along the white dashed line within the cell shown on the left. The cell was illuminated five times (blue arrows above the kymograph) every 10 min. ( e ) (Left) A HeLa cell co-expressing optoTrkB and R-GECO1 was exposed to whole-cell () or local ( and ) light stimulation. The stimulated areas are outlined with white dashed lines. (Right) Time-lapse, pseudocolored surface intensity plots. Local stimulation is marked with arrows. Axis labelled ‘I’ represents intensity. Scale bar, 20 μm. ( f ) Selective induction of Ca 2+ transients. HeLa cells transfected with R-GECO1 or cotransfected with optoTrkB and R-GECO1 (arrowheads) were co-cultured (mixed population) and simultaneously exposed to blue-light pulses. Time courses of R-GECO1 responses are represented by ratio images. Scale bar, 50 μm. Full size image We next examined the subcellular resolution and spatial selectivity of optically activated TrkB signalling. Whole-cell illumination, in which light stimulation is confined to the whole area of a single cell, caused an increase in [Ca 2+ ] i simultaneously throughout the cell ( Fig. 3e , top). In contrast, when blue-light pulses were delivered locally, Ca 2+ signals were generated precisely from at each edge of a single cell and then propagated ( Fig. 3e , middle and bottom). Thus, we were able to achieve fine spatial control of TrkB signalling. Moreover, in a mixed cell population containing HeLa cells with and without optoTrkB expression, global photostimulation, in which an illumination area covers more than one cell, selectively increased [Ca 2+ ] i only in cells expressing optoTrkB ( Fig. 3f and Supplementary Movie 2 ), demonstrating cell-specific modulation of signalling. In addition to Ca 2+ signal, an investigation of endogenous ERK activity demonstrated that TrkB signalling activity was light-controllable. Upon exposure of a population of optoTrkB-transfected HeLa cells to a 1-min global illumination (470 nm) using a blue LED array, phospho-ERK level was increased approximately fivefold after 5 min and declined after 25 min ( Supplementary Fig. 7 ). A subsequent, second stimulation applied after a 25-min interval gave rise to a second increase in phospho-ERK ( Supplementary Fig. 7 ), confirming that endogenous signalling activity in a group of optoTrkB-expressing cells can be reversibly and synchronously modulated by light. Light-induced neurite outgrowth by sustaining ERK activity One of the prominent trophic effects of neurotrophins in Trk-expressing neuronal cells is promotion of neurite outgrowth. Nerve growth factor-induced neurite outgrowth in the rat pheochromocytoma cell line, PC12, has been extensively studied and characterized in this context [20] , [21] . Nerve growth factor treatment of PC12 cells, which endogenously express TrkA, induces neuronal differentiation, a process in which sustained activation of ERK is essential [20] , [21] . Because TrkA and TrkB signalling pathways involve similar signalling proteins and PC12 cells expressing TrkB respond to BDNF by extending their neurites [22] , we exploited this morphological response as a functional readout to evaluate whether light stimulation could mimic the biological effects of BDNF/TrkB signalling in optoTrkB-transfected PC12 cells. We first optimized illumination conditions by varying illumination duration and ISIs based on the light-triggered ERK dynamics in HeLa ( Supplementary Figs 3 and 4 ) at a constant laser power (5.5 μW). Exposure of PC12 cells transfected with optoTrkB to a single 5-s illumination with blue LED (470 nm) led to a rapid increase in the level of active ERK within 5 min, which diminished thereafter ( Fig. 4a ); these results paralleled those obtained in HeLa cells ( Supplementary Figs 3 and 4 ). Notably, exposure to repetitive illumination (5 s on/5 min off) induced a high level of active ERK that was sustained for at least 4 h ( Fig. 4a ). Thus, we could produce long-duration ERK activity by stimulating optoTrkB-mediated signalling using a repetitive, alternating light-ON/light-OFF protocol. 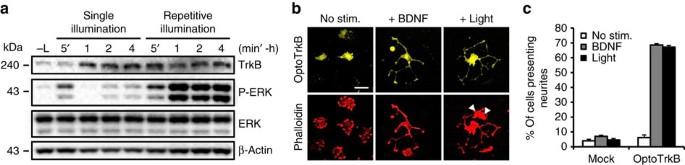Figure 4: Induction of neurite outgrowth by light-triggered, sustained ERK activity. (a) Sustained activation of ERK by light. Serum-starved (24 h) optoTrkB-transfected PC12 cells were exposed to a single 5-s irradiation and left in the dark (single illumination) or to repetitive 5-s irradiations every 5 min (repetitive illumination) using a blue LED array (470 nm and 5.5 μW). ERK activity was examined at the indicated times. β-Actin was included as a protein loading control. (b) Representative images of optoTrkB-transfected (upper panel) and phalloidin-stained (lower panel) PC12 cells. Serum-starved (24 h) optoTrkB-transfected PC12 cells were unstimulated (no stim.) or stimulated with BDNF (50 ng ml−1) or with a 5-s ON/5-min OFF illumination protocol using a blue LED array for an additional 24 h. Phalloidin-stained cells marked with white arrowheads (on ‘+Light’ panel) denote non-transfected PC12 cells. Scale bar, 50 μm. (c) Quantification of neurite outgrowth. Non-transfected (mock) and optoTrkB-transfected PC12 (optoTrkB) cells treated as described inbwere scored for the presence of neurites. Cells presenting neurites were defined as those with at least one neurite more than one cell–body diameter in length. Results are expressed as the percentage of neurite-bearing cells in the total number of counted cells. At least 100 cells were counted in each experiment and data are presented means±s.e. of three independent experiments. Figure 4: Induction of neurite outgrowth by light-triggered, sustained ERK activity. ( a ) Sustained activation of ERK by light. Serum-starved (24 h) optoTrkB-transfected PC12 cells were exposed to a single 5-s irradiation and left in the dark (single illumination) or to repetitive 5-s irradiations every 5 min (repetitive illumination) using a blue LED array (470 nm and 5.5 μW). ERK activity was examined at the indicated times. β-Actin was included as a protein loading control. ( b ) Representative images of optoTrkB-transfected (upper panel) and phalloidin-stained (lower panel) PC12 cells. Serum-starved (24 h) optoTrkB-transfected PC12 cells were unstimulated (no stim.) or stimulated with BDNF (50 ng ml −1 ) or with a 5-s ON/5-min OFF illumination protocol using a blue LED array for an additional 24 h. Phalloidin-stained cells marked with white arrowheads (on ‘+Light’ panel) denote non-transfected PC12 cells. Scale bar, 50 μm. ( c ) Quantification of neurite outgrowth. Non-transfected (mock) and optoTrkB-transfected PC12 (optoTrkB) cells treated as described in b were scored for the presence of neurites. Cells presenting neurites were defined as those with at least one neurite more than one cell–body diameter in length. Results are expressed as the percentage of neurite-bearing cells in the total number of counted cells. At least 100 cells were counted in each experiment and data are presented means±s.e. of three independent experiments. Full size image Adopting this illumination protocol, we stimulated optoTrkB-transfected PC12 cells with blue-light pulses for 24 h and examined neurite outgrowth after phalloidin staining. In the absence of a stimulus, the morphology of undifferentiated PC12 cells was not affected by the expression of optoTrkB ( Fig. 4b,c ). In addition, repetitive illumination did not promote neurite formation in non-transfected PC12 cells ( Fig. 4b , white arrowheads; and Fig. 4c , mock). However, 24-h repetitive irradiation markedly induced neurite extensions in optoTrkB-transfected PC12 cells, producing an effect comparable to that of BDNF stimulation ( Fig. 4b,c ). The neurite outgrowth responses were affected by light intensity; the total neurite length and the length of the longest neurite was increased in an illumination dose-dependent manner ( Supplementary Fig. 8 ). In addition, we also monitored light-driven neurite outgrowth by using real-time, live-cell imaging ( Supplementary Movie 3 ). In line with the staining data, repetitive light stimulation caused morphological changes in optoTrkB-expressing PC12 cells that did not occur in the absence of illumination. Taken together, these results indicate that BDNF/TrkB signalling activity was recapitulated by light control of optoTrkB. More importantly, they also suggest that optoTrkB expression, which, in theory, could lead to receptor auto-activation [23] , did not spontaneously cause any marked biological consequences; expression of these receptors was functionally effective only when coupled with light stimulation. Functional expression of optoTrkB in primary neurons Finally, we examined optoTrkB performance in cultured rat hippocampal neurons. In a neuron at 7 DIV, which was cotransfected with optoTrkB and mCh-PH AKT1 , blue-light irradiation triggered rapid translocation of mCh-PH AKT1 to the plasma membrane in the soma ( Supplementary Fig. 9a–c ), thereby demonstrating optoTrkB functionality. During this observation, we also found that filopodia- and lamellipodia-like structures (yellow arrows and blue arrowheads, respectively) were formed in the perisomatic region of the irradiated neuron ( Supplementary Fig. 9d ). Given that BDNF/TrkB signalling activity has shown to drive an activity-dependent synapse formation process [24] , in part by inducing filopodia and spine formation, and based on our observation, we next investigated light-induced filopodia formation using optoTrkB. For the visualization of the filopodial dynamics, we co-expressed mCherry-tagged LifeAct (mCh-LifeAct), which stains filamentous actin [25] . At first, live-cell imaging of hippocampal neurons overexpressing wild-type TrkB (TrkB-mCit) showed that BDNF (100 ng ml −1 ) treatment induced the filopodia formation ( Supplementary Fig. 10a–c ). The number of filopodia in neuritic processes was increased by nearly twofold after a 10-min administration of BDNF and plateaued thereafter ( Supplementary Fig. 10c ). Based on this, we next examined optoTrkB- and TrkB-mCit-transfected neurons after light and BDNF stimulation, respectively, for 30 min. OptoTrkB expression per se did not augment neuronal filopodia density in the dark, comparable to that caused by TrkB-mCit expression in the absence of BDNF ( Supplementary Fig. 11a–c ). However, repetitive or continuous illumination induced a significant increase in the number of filopodia ( Supplementary Fig. 11c ). In addition, focal photostimulation elicited a spatially restricted formation of filopodia ( Fig. 5a–c ). Time-lapse imaging of a single neuron expressing optoTrkB and mCh-LifeAct revealed that when exposed to a localized irradiation, the number of filopodia was increased only within the stimulated area but not in nearby non-stimulated area ( Fig. 5b,c ). Taken together, these results demonstrated an optical control of filopodial formation using optoTrkB in a temporally precise and spatially specific fashion. 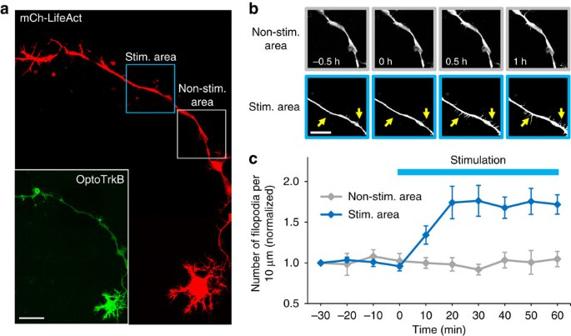Figure 5: Optical control of local filopodia formation in a hippocampal neuron expressing optoTrkB. (a) A hippocampal neuron (DIV 7) transfected with optoTrkB and mCh-LifeAct. Scale bar, 50 μm. (b) Time-lapse images showing non-stimulated (non-stim., marked by grey box ina) and stimulated (stim., marked by blue box ina) areas in the neuron shown ina. The stimulated area was exposed to three 0.5-s pulses of blue light (6.5 μW) every 30 s for 1 h. Yellow arrows in the stimulated area highlight the newly formed filopodia. (c) Quantification of the number of filopodia. The number of filopodia in neuritic processes per 10 μm was calculated at each time points and normalized to baseline (at −30 min). Error bars, ±s.e.m. (n=7). The blue bar in the graph indicates stimulation period. Figure 5: Optical control of local filopodia formation in a hippocampal neuron expressing optoTrkB. ( a ) A hippocampal neuron (DIV 7) transfected with optoTrkB and mCh-LifeAct. Scale bar, 50 μm. ( b ) Time-lapse images showing non-stimulated (non-stim., marked by grey box in a ) and stimulated (stim., marked by blue box in a ) areas in the neuron shown in a . The stimulated area was exposed to three 0.5-s pulses of blue light (6.5 μW) every 30 s for 1 h. Yellow arrows in the stimulated area highlight the newly formed filopodia. ( c ) Quantification of the number of filopodia. The number of filopodia in neuritic processes per 10 μm was calculated at each time points and normalized to baseline (at −30 min). Error bars, ±s.e.m. ( n =7). The blue bar in the graph indicates stimulation period. Full size image We also tested the effects of pulsatile optoTrkB activation on the neurite outgrowth process in young hippocampal neurons. To this end, we expressed optoTrkB in freshly dissociated hippocampal neurons and stimulated them with BDNF (100 ng ml −1 ) or light (25 μW) from DIV 1 to DIV 3 (for 48 h), during which neuronal polarity is spontaneously established [26] (control; Supplementary Fig. 12a ). Blue-light illumination, as well as BDNF incubation, significantly increased the total neurite length ( Supplementary Fig. 12b ) and the number of branch points ( Supplementary Fig. 12c ) in young hippocampal neurons. BDNF incubation caused more prominent effects on neurite outgrowth than light stimulation, likely through the binding of BDNF to endogenous TrkB or p75 neurotrophic receptors [19] . In addition to validating its functionality in primary neurons, we also monitored vesicular transport of optoTrkB receptor. Upon ligand binding at the axonal terminal, TrkB receptor is internalized and delivered in the retrograde direction, and thereby initiates retrograde signalling [27] . Therefore, BDNF signalling in neurons relies on proper transport of its TrkB receptor [28] . We compared the axonal transport of TrkB-mCit and optoTrkB in hippocampal neurons ( Fig. 6a,b ). A few vesicles were immobile (white asterisks) but most of them were mobile (arrows). And similarly as TrkB-mCit ( Fig. 6a ), optoTrkB receptors were actively retrogradely transported along the axon ( Fig. 6b ), demonstrating that the modified TrkB receptor was able to be internalized and transported in hippocampal neurons. 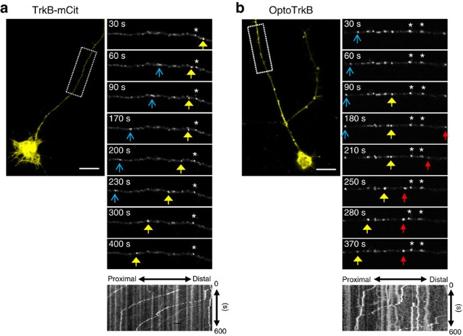Figure 6: Dynamic movements of wild-type TrkB and optoTrkB in axons. (a,b) Hippocampal neurons (DIV 8) were transfected with (a) TrkB-mCit or (b) optoTrkB, and movement of them were monitored along the axons (the longest neurite among others) by capturing images every 5 s for 10 min. The white boxes in representative TrkB-mCit and optoTrkB images indicate the area shown on right of each of them. The stationary and moving vesicles are marked by asterisks and arrows, respectively, and arrows with different colours indicate different individual vesicles. Kymographs show movement of TrkB-mCit and optoTrkB from a distal to proximal region of the axons, indicating retrograde transport. Scale bars, 20 μm. Figure 6: Dynamic movements of wild-type TrkB and optoTrkB in axons. ( a , b ) Hippocampal neurons (DIV 8) were transfected with ( a ) TrkB-mCit or ( b ) optoTrkB, and movement of them were monitored along the axons (the longest neurite among others) by capturing images every 5 s for 10 min. The white boxes in representative TrkB-mCit and optoTrkB images indicate the area shown on right of each of them. The stationary and moving vesicles are marked by asterisks and arrows, respectively, and arrows with different colours indicate different individual vesicles. Kymographs show movement of TrkB-mCit and optoTrkB from a distal to proximal region of the axons, indicating retrograde transport. Scale bars, 20 μm. Full size image Light control of cell signalling offers an unprecedented opportunity to interrogate the spatial and temporal dynamics of intracellular signalling circuits [29] . Moreover, it also opens new avenues for investigating causal links between biochemical signalling and animal behaviour [3] . By simply combining a light-sensitive homo-interaction module with a receptor-dimerization system—and without considerable engineering—we have added new single-component optogenetic tools, optoTrk receptors ( Fig. 1b,c and Supplementary Fig. 2 ), to the existing light-controllable toolkit. OptoTrk receptors provoke upregulation of canonical Trk pathways in response to blue-light exposure ( Fig. 1c and Supplementary Fig. 2 ), demonstrating that receptor modification, the addition of PHR domain and mCitrine ( Fig. 1b ) does not alter signalling activity of native receptors. In addition, a photoactivatable form of TrkB mutated at Tyr-816 (Y816F) [30] (TrkB Y816F -PHR-mCit), which is the PLCγ1-binding site, failed to elevate [Ca 2+ ] i after blue-light stimulation ( Supplementary Fig. 13 ), further supporting that specific tyrosine phosphorylation, but not the C-terminally fused domains, influences the binding of proteins that are recruited at TrkB receptor. The Trk receptors, like most RTKs, are activated by ligand-induced receptor dimerization. Accordingly, overexpression of them are prone to receptor auto-activation in the absence of stimulus [23] . Indeed, for example, a modest induction of optoTrkB activation in the dark state, as demonstrated by an increase in ERK phosphorylation without illumination, was evident in HeLa cells ( Supplementary Figs 3a and 5a ), which may limit the utility of optoTrkB. However, we also observed that first, TrkB-mCit expression in HeLa cells was also shown to induce ERK phosphorylation in the absence of BDNF treatment ( Supplementary Fig. 4c ); and second, no significant increase in background ERK activity was observed in PC12 cells regardless of optoTrkB expression level ( Supplementary Fig. 14 ). Thus, these results suggest that not optoTrkB expression per se , but cell lines for its expression was responsible for the background signal activity. A light-inducible protein–protein interaction with fast association and dissociation kinetics has the benefits of temporally precise control of cell signalling. Moreover, a genetically encoded dimerization system based on light-mediated protein homo-interactions is highly favourable compared with that based on protein hetero-interactions. The photoactivatable receptors in this study, optoTrks, are based on PHR domain of cryptochrome 2 as a single light-responsive dimerizer. And upon blue-light exposure, optoTrk(B) rapidly (within seconds) and transiently (for a few minutes) activates corresponding signalling pathways ( Fig. 2 ) without the need for exogenous cofactors, thus PHR meets the requirements for an ideal optogenetic dimerizer. The light-dependent homo-interaction property of PHR described here has been recently reported, showing that PHR can be oligomerized and form clusters by blue-light illumination in mammalian cells [31] . Thus, as suggested [31] , our results further support that PHR can be harnessed as a single light-sensitive module to induce protein–protein interaction and can be adapted to a broad range of signalling molecules, including other RTK families. Our light-dependent strategy offers several advantages over conventional ligand-based or pharmacological approaches, including those use organic compounds (such as CIDs) and engineered receptors [9] , [10] , [11] , for the control of receptor signalling. First, it has high temporal resolution, producing faster signalling responses ( Fig. 2 ). Second, it is fully reversible in the minute timescale and enables precisely controlled repetitive activation ( Fig. 3a–d ). Third, it allows spatially restricted activation of cell signalling ( Figs 3e and 5 ). Fourth, it lacks off-target effects and has cell-type specificity ( Fig. 3f ). In addition, it causes induction of transient and sustained protein activity by a single and a repetitive illumination, respectively ( Supplementary Fig. 4 and Fig. 4a ), thus providing a simple means to manipulate the functional duration of signalling. In summary, optoTrkB enables versatile control of TrkB signalling and thus allows quantitative investigation of spatiotemporal signalling dynamics in vitro and in vivo . Moreover, it recapitulates BDNF/TrkB signalling activity in response to light, thereby possessing beneficial properties from both cell biological and therapeutic perspectives [19] . Further engineering of optoTrk receptors to a truncated form to prevent endogenous ligand binding [10] could make this tool readily applicable to in vivo systems. Plasmid construction TrkB cDNA was provided by K. Kaibuchi (Nagoya University, Nagoya), and TrkA, TrkB Y816F and TrkC cDNAs were provided by L.C. Schecterson (University of Washington, Seattle, WA). CIBN-pmGFP was provided by C.L. Tucker (University of Colorado Denver, Denver, CO). For efficient mammalian expression, the PHR-coding sequence [7] was codon-optimized (here referred to as PHR) and listed in Supplementary Fig. 15 . To construct chimeric TrkB, we first generated PHR-mCitrine by inserting Nhe I/ Age I-restricted PHR into the corresponding sites ( Nhe I/ Age I) of pmCitrine-C1 (Clontech) and CIBN-mCerulean by inserting Nhe I/ Age I-restricted CIBN from CIBN-pmGFP into the corresponding sites ( Nhe I/ Age I) of pmCerulean-C1 (Clontech). Next, Nhe I/ Bam HI-restricted TrkB, amplified by polymerase chain reaction (PCR) from TrkB cDNA using TrkB-F (5′-ggaaaa gctagc ATGTCGCCCTGGCCGAGGTGG-3′) and TrkB-R (5′-ggaaaa ggatcc CCTAGGATGTCCAGGTAGACGG-3′) primers was cloned into the corresponding sites ( Nhe I/ Bam HI) in the multicloning site (MCS) of pEGFP-N1 (Clontech). The resulting TrkB-EGFP was further restricted with Nhe I/ Bsr GI and cloned into the corresponding sites ( Nhe I/ Bsr GI) of pEGFP-C1 (Clontech) to yield TrkB-EGFP-MCS. Finally, 5′ blunt-ended and 3′ Mlu I-restricted PHR-mCitrine, PCR-amplified from the PHR-mCitrine vector using PHR-F (5′-tcgccaccATGAAGATGGACAAAAA-3′) and Mlu I-R (5′-gaa acgcgt TTACTTGTACAGCTCGTCCATGC-3′) primers, or 5′ blunt-ended and 3′ Mlu I-restricted CIBN-mCerulean, PCR-amplified from CIBN-mCerulean vector using CIBN-F (5′-tcgccaccATGAATGGAGCTATAGGAGGTGA-3′) and Mlu I-R primers, were inserted into TrkB-EGFP-MCS restricted with Age I, filled in using Klenow fragment and further restricted with Mlu I. The resulting constructs, TrkB-PHR-mCitrine (optoTrkB) and TrkB-CIBN-mCerulean, encode full-length TrkB fused to PHR-mCitrine and CIBN-mCerulean, respectively, via a linker derived from pEGFP-N1 (DPPVAT). TrkB-CIBN-mCitrine was cloned following the same procedures described above, and TrkB-mCitrine was constructed by excising PHR from TrkB-PHR-mCitrine by using Age I and re-ligating it. TrkB-PHR D387A -mCitrine was generated by site-directed mutagenesis, as described [32] , using Age I-PHR-F (5′-ggatcc accggt cgccaccATGA-3′), (D387A)PHR-R (5′-CCAAGTCGGCG G CGAGAAGGGTA-3′), (D387A)PHR-F (5′-TACCCTTCTCG C CGCCGACTTGG-3′) and PHR- Age I-R (5′-cggcagccc accggt CGCCA-3′) primers. TrkB Y816F -PHR-mCitrine was constructed by replacing TrkB from TrkB-PHR-mCitrine with PCR-amplified TrkB Y816F using BamH I and Nhe I restriction sites. TrkA-PHR-mCitrine (optoTrkA) and TrkC-PHR-mCitrine (optoTrkC) were constructed by inserting TrkA and TrkC cDNAs in place of the TrkB of optoTrkB using In-Fusion HD Cloning Kits (Clontech). The CMV (cytomegalovirus) promoter of optoTrkB was replaced by PGK (phosphoglycerate kinase 1) promoter of pPGK-Cre-bpA (plasmid 11543, Addgene) by Ase I and Nhe I digestion. ERK-mCherry was constructed by transferring the coding region of an Erk1 entry clone, created using Alliance for Cellular Signaling (AfCS) vector pEX_EF1_Erk1-YFP (AfCS barcode: A05XP002A1NK), into an mCherry expression vector using LR Clonase (Invitrogen). mCherry-PH AKT1 has been described previously [18] and the R-GECO1 expression vector (CMV-R-GECO1) is available from Addgene (plasmid 32444). mCherry-LifeAct was constructed by replacing GFP from GFP-LifeAct [25] to mCherry by using Nhe I and BsrG I restriction sites. Reagents Recombinant human BDNF was purchased from R&D Systems (cat. no. 248-BD) and reconstituted in sterile phosphate-buffered saline (PBS). K252a (cat. no. K1639) and U73122 (PLC inhibitor; cat. no. U6756) were purchased from Sigma-Aldrich and dissolved in dimethyl sulfoxide (DMSO). LY294002 (PI3K inhibitor) was obtained from LC Laboratories (cat. no. L-7962) and dissolved in DMSO. PD0325901 (MEK inhibitor) was obtained from Cayman Chemical (cat. no. 13034) and dissolved in DMSO. Poly- D -lysine hydrobromide was obtained from Sigma-Aldrich (cat. no. P6407). Cell culture and transfection HeLa (American Type Culture Collection, ATCC) cells were cultured in Dulbecco’s modified Eagle’s medium (DMEM; cat. no. E15-843; PAA Laboratories GmbH) supplemented with 10% fetal bovine serum (FBS; cat. no. A12617; Gibco, Invitrogen) at 37 °C in a humidified 10% CO 2 atmosphere. The PC12 subline, Neuroscreen-1 (here referred to as PC12; Cellomics) [33] , was provided by T. Meyer (Stanford University, Stanford, CA) and cultured in F-12K media (cat. no. 10-025-CV; Cellgro) supplemented with 15% horse serum (cat. no. 16050-122; Gibco, Invitrogen) and 5% FBS at 37 °C and 5% CO 2 . Cells were transfected using a Microporator (Neon Transfection System; Invitrogen) according to the manufacturer’s instructions. In brief, for live-cell imaging, 2 × 10 5 HeLa or PC12 cells were mixed with a total of 0.6 μg DNA (0.3 μg each DNA in cotransfection experiments), electroporated, diluted 1:5 and seeded into a 96-well glass-bottom microplate (cat. no. MGB096-1-2-LG-L; Matrical Bioscience). For immunoblot analysis, 5 × 10 5 HeLa or 2 × 10 6 PC12 cells, transfected by electroporation with a total of 6 μg DNA, were seeded per well of a six-well plate. Preparation and transfection of hippocampal neurons E18 pregnant Sprague–Dawley female rats were prepared for hippocampal cultures. All experimental procedures were approved by the Animal Ethic Committee at the Korea Advanced Institute of Science and Technology (KAIST; Daejeon, Korea). In brief, embryos were obtained from the rats and then placed into Hank's Balanced Salt Solution (HBSS) (cat. no. 14185-052; Gibco)–HEPES (10 mM; cat. no. 15630-080; Gibco) solution. Hippocampi were dissected from the embryos and incubated in 0.25% trypsin for 25 min at 37 °C with tapping every 5 min. Hippocampi were washed for three times with HBSS–HEPES, and triturated with a fire-polished Pasteur pipette. Tissues were dissociated after 10–20 trituration, and neurons were immediately plated in pre-equilibrated dishes or plates coated with 1 mg ml −1 poly-L-lysine (cat. no. P2636; Sigma) in plating medium. The plating medium consisted of Neurobasal medium (cat. no. 21103-049; Gibco) supplemented with 2% FBS, 2% B-27 (cat. no. 17504-044; Gibco), 2% glutamax (cat. no. 35050-061; Gibco) and 2% penicillin–streptomycin (cat. no. 15140-122; Gibco). The neurons were incubated at 37 °C in a humidified 5% CO 2 atmosphere. Plating medium were replaced with maintaining medium (plating medium without FBS) within 6–24 h. Neurons were transfected with LipofectamineLTX and plus reagent (Invitrogen) in Opti-MEM (Invitrogen) following manufacturer’s instruction. In brief, total 0.5 μg of DNA was incubated with 0.5 μl of plus reagent in 100 μl of Opti-MEM for 5 min, and then 0.5 μl LipofectamineLTX was added to the mixture. After 20 min incubation at room temperature, 20 μl from 100 μl mixture was dropped into a well of a 96-well microplate where the medium was completely replaced to 100 μl of the new maintaining medium. The medium was then replaced to the kept conditioned medium after 45 min. Live-cell imaging, photostimulation and data acquisition Cells were imaged 24 h after transfection. Before monitoring ERK and AKT activity, transfected HeLa cells were serum-starved for 6 h. Just before imaging ERK, AKT and Ca 2+ activity, the medium was replaced with Dulbecco’s PBS containing glucose (cat. no. 14287080; Invitrogen). Neurite outgrowth was observed by imaging transfected PC12 cells in serum-free medium (F-12K). Live-cell imaging was performed using a Nikon A1R confocal microscope (Nikon Instruments) mounted onto a Nikon Eclipse Ti body and equipped with CFI Plan Apochromat VC objectives (60 × /1.4-numerical aperture (NA) oil or 40 × /0.95-NA air; Nikon) and a Chamlide TC system (maintained 37 °C and 10 or 5% CO 2 ; Live Cell Instrument, Inc., Korea). mCerulean, GFP, mCitrine and mCherry images (512 × 512 pixels, 72.7 μm 2 ) were taken using 457-, 488-, 514- and 561-nm laser lines, respectively. A built-in photo activation illumination unit was used to excite the illumination volume (generally confined to a single cell except for the experiments shown in Fig. 3f and Supplementary Movies 2 and 3 ) with 488-nm light during live-cell imaging. The 488-nm laser intensity used for photostimulation (6.5 μW per 72.7 m 2 =1.27 mW cm −2 ; here denoted simply as 6.5 μW) was measured right above the objective. The images were analysed with Nikon imaging software (NIS-element AR 64-bit version 3.10; Laboratory Imaging) and MetaMorph software (version 7.6.0.0; MDS Analytical Technologies). Electronics An optical power meter (cat. no. 8230E; ADCMT, Japan) was used to measure blue-light intensity. We used two types of illumination devices consisting of 24 and 96 blue LEDs (cat. no. PP465-8L63-ESESBI; Photron, Korea) mounted on a customized array (Live Cell Instrument, Inc.; Supplementary Fig. 16 ). For the 24 LED array, each set of four LEDs was positioned at the centre of each well of a six-well plate. The LEDs emitted an equal intensity blue light onto cells in a six-well plate (5.5 μW, measured 1 cm from the LEDs) and the light pulses were controlled using a digital time switch (cat. no. TR 611 top2; Theben). The 96 LEDs were positioned to fit into wells of a 96-well glass-bottom microplate, and eight LEDs in each column were simultaneously controlled using Micro-manager software (version 1.4.15) to allow independent control of 12 columns. Immunoblot analysis Whole-cell lysates were prepared in the dark using PRO-PREP solution (cat. no. 17081; iNtRON Biotechnology) and 20 μg of total protein was resolved on a NuPAGE Novex 4–12% Bis-Tris gel (Invitrogen). Proteins were transferred to a nitrocellulose membrane using an iBlot Transfer Stack and iBlot Gel Transfer Device (Invitrogen) according to the manufacturer’s instructions. The membrane was immunoblotted by incubating first with primary rabbit anti-TrkB (1:1,000; cat. no. 4606; Cell Signaling Technology), rabbit anti-phospho-Erk1/2 (1:1,000; cat. no. 9101; Cell Signaling Technology), rabbit anti-Erk1/2 (1:1,000; cat. no. 9102; Cell Signaling Technology), rabbit anti-β-tubulin (1:1,000; cat. no. 04-1049; Millipore) and/or mouse anti-β-actin (1:1,000; cat. no. A5316; Sigma) antibodies, and then with horseradish peroxidase conjugated anti-rabbit immunoglobulin (IgG-HRP) (1:3,000; cat. no. NA934V; GE Healthcare) or anti-mouse IgG-HRP (1:3,000; cat. no. sc-2005; Santa Cruz Biotechnology) secondary antibodies, as appropriate, using standard procedures. Proteins were visualized using SuperSignal West Pico Chemiluminescent Substrate (cat. no. 34080; Thermo Scientific) and a ChemiDoc MP system (Bio-Rad). For the blots shown in Supplementary Figs 4 and 7 , following secondary antibodies were used: goat-anti-mouse IR Dye 800CW (1:3,000; cat. no. 926-32210; LI-COR) or goat-anti-rabbit IR Dye 600CW (1:3,000; cat. no. 626-68071; LI-COR). These blots were scanned by Odessey CLx Infrared Imaging system (LI-COR). Densitometric analysis was carried out on the immunoblots using MetaMorph software. Uncropped gel scans of all western blots in this paper were presented in Supplementary Fig. 17 . Neurite outgrowth assay OptoTrkB-transfected PC12 cells in poly- D -lysine-coated 96-well plates were serum-starved for 24 h and either left unstimulated, treated with BDNF (50 ng ml −1 ) or exposed to pulsatile illumination (5-s irradiation every 5 min, 470 nm, 5.5 μW) administered with a blue LED array for an additional 24 h in serum-free media at 37 °C in a humidified 5% CO 2 environment. All the samples were kept in the dark for the duration. Cells were fixed by incubating with a 4% methanol-free formaldehyde solution in PBS (cat. no. 28908; Thermo Scientific) and permeabilized with 0.1% Triton X-100 in PBS. Filamentous actin was stained with Alexa Fluor 594-conjugated phalloidin (cat. no. A12381; Invitrogen) and cells were imaged using a confocal microscope. The number of neurite-presenting cells, the total neurite length and the length of the longest neurite were measured and analysed with ImageJ software ( http://rsbweb.nih.gov/ij/ ). Freshly dissociated hippocampal neurons (DIV 0) were transfected with optoTrkB and after 24 h, they were either non-stimulated or stimulated with BDNF (100 ng ml −1 ) or light pulses (25 μW) at 37 °C in a humidified 5% CO 2 environment for additional 48 h. All the samples were kept in the dark for the duration. Cells were fixed by incubating with a 4% methanol-free formaldehyde solution in PBS and imaged using a confocal microscope. The total neurite length and the number of branch points per cell were measured and analysed using MetaMorph software. Filopodia formation assay For the live-cell imaging, neurons at DIV 5–7 were transfected with TrkB-mCitrine or optoTrkB and mCherry-LifeAct. After 24 h, they were treated with BDNF (100 ng ml −1 ) or light pulses (6.5 μW) for 1 h and images were taken using a confocal microscope. For the analysis of fixed samples, neurons at DIV 5 were transfected with TrkB-mCitrine or optoTrkB and exposed to BDNF (100 ng ml −1 ) or light pulses using a blue LED array (25 μW) for 30 min, respectively. Cells were fixed, permeabilized, stained with Alexa Fluor 594-conjugated phalloidin, and then imaged using a confocal microscope. Filopodia were defined as any protrusion under 10 μm in length. The number of filopodia per 10 μm were measured and analysed using Nikon imaging software. How to cite this article: Chang, K.-Y. et al . Light-inducible receptor tyrosine kinases that regulate neurotrophin signalling. Nat. Commun. 5:4057 doi: 10.1038/ncomms5057 (2014).